Biogeography and habitat modelling of high-alpine bacteria Soil microorganisms dominate terrestrial biogeochemical cycles; however, we know very little about their spatial distribution and how changes in the distributions of specific groups of microbes translate into landscape and global patterns of biogeochemical processes. In this paper, we use a nested sampling scheme at scales ranging from 2 to 2,000 m to show that bacteria have significant spatial autocorrelation in community composition up to a distance of 240 m, and that this pattern is driven by changes in the relative abundance of specific bacterial clades across the landscape. Analysis of clade habitat distribution models and spatial co-correlation maps identified soil pH, plant abundance and snow depth as major variables structuring bacterial communities across this landscape, and revealed an unexpected and important oligotrophic niche for the Rhodospirillales in soil. Furthermore, our global analysis of high-elevation soils from the Andes, Rockies, Himalayas and Alaskan range shows that habitat distribution models for bacteria have a strong predictive power across the entire globe. Despite the known importance of microorganisms to the maintenance of the Earth's biogeochemical cycles [1] , [2] , the relationship between the ecological niche of microbial groups and the culture-independent identification of their presence in the environment is poorly understood [3] , [4] , [5] . This is because of lack of resolution in data collected using traditional methods, which obscures the identification of potentially important groups across a landscape [3] . However, Ettema and Wardle [3] point out that, given enough data, 'spatial variability is the key, rather than the obstacle, to understanding the structure and function of soil biodiversity'. Previous studies have shown that there are spatial patterns to microorganisms [6] , [7] , [8] , [9] , [10] and that some coarse-scale taxonomic groups (at the phylum or division level) show strong correlation with environmental parameters; for example, Acidobacteria are negatively correlated with soil pH, whereas Proteobacteria are positively correlated with pH [11] , [12] . However, groups such as the Acidobacteria and Proteobacteria are extremely large and functionally diverse; for example, Proteobacteria encompass almost all known microbial physiologies ranging from phototrophs to heterotrophs to chemoautotrophs, and recent studies indicate that the Acidobacteria may be equally metabolically diverse [13] . Thus, we gain very little information about the biogeochemistry of a specific system or of the global biosphere by knowing the spatial distribution of such large taxonomic groups. Similarly, we still have only a rudimentary understanding of the local spatial scale at which soil microbes and soil biogeochemical parameters are distributed. Furthermore, matching the relative abundance patterns of specific microbial taxa and biogeochemistry at both local and global scales has remained an elusive task. Our study makes use of recent advances in high-throughput sequencing, bioinformatics and biogeochemical methods [14] , [15] , [16] , [17] , [18] , [19] to map the co-occurrence of microbial groups with biogeochemical soil properties across a highly heterogeneous, high-elevation landscape near the continental divide in the Rocky Mountains of Colorado, USA [20] , [21] , [22] . On the basis of our previous study of the spatial autocorrelation of soil biogeochemical properties [22] , we collected 160 soil samples in a nested sampling scheme. This sampling scheme allowed us to determine spatial variation in microbial diversity (a random subset of 85 samples was pyrosequenced for the 16S gene) and its relationship to 21 soil biogeochemical properties at scales from 2 to 2,000 m in Colorado. These analyses were essential for obtaining spatially explicit, landscape habitat distributions (models based on co-variation of relative abundance with biogeochemistry) for bacterial community members, which were tested at a global scale by sampling similar soils in the Colorado Rockies, Himalayas, Andes and Alaskan range (Sanger clone libraries of the 16S gene). In this study, we show that bacterial communities have significant spatial autocorrelation at distances up to 240 m; however, beyond that distance, community composition does not display significant spatial autocorrelation. In addition, the dominant bacterial clades from the landscape-scale survey display strong co-variation with biogeochemical parameters, such that their relative abundances across the globe are predictable using habitat distribution models. Landscape patterns in bacterial community relatedness The first step in assessing habitat distributions for bacteria was to determine whether there was a significant spatial pattern to their distribution across the landscape (see Fig. 1 for sampling design). We used Unifrac phylogenetic analysis [18] , [19] to show that there was a significant change in community relatedness with increasing distance between any two samples across the landscape ( n = 85, P = 0.001, Mantel test) up to a maximum autocorrelation distance of 240 m ( Fig. 2 ). However, the change in community relatedness up to this scale was somewhat small (change in UniFrac distance over 240 m = 0.03), perhaps indicating that only a subset of the total bacterial community is changing across the landscape. In contrast, beyond 240 m, there is a random scatter of data around the plateau value that is equal to the average community relatedness among all samples (see inset to Fig. 2 ); thus, at distances greater than 240 m, it is just as likely to find a closely related community as it is to find a distantly related community. 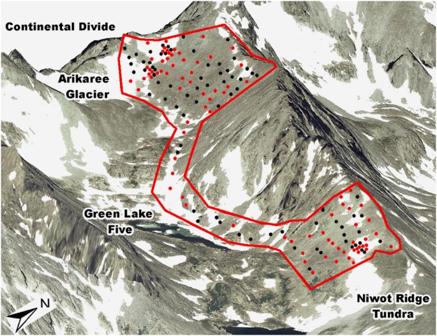Figure 1: Landscape sampling scheme. Satellite image of the sampling area in Green Lakes Valley, Colorado (40°3′24″N 105°37′30″W). Black dots indicate sampling locations and red dots indicate the samples that were sequenced for bacterial community composition. The distance between the farthest two samples was 2 km. Figure 1: Landscape sampling scheme. Satellite image of the sampling area in Green Lakes Valley, Colorado (40°3′24″N 105°37′30″W). Black dots indicate sampling locations and red dots indicate the samples that were sequenced for bacterial community composition. The distance between the farthest two samples was 2 km. 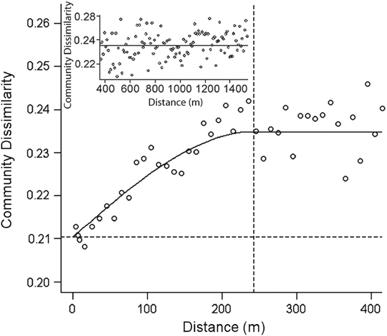Figure 2: Community-level spatial autocorrelation semivariogram. A semivariogram plot of the decay in community similarity (as measured by the UniFrac community dissimilarity metric on theyaxis) with increasing distance between samples. A UniFrac value of 1 indicates no shared community members between two samples and a value of 0 indicates 100% shared community members. The solid line is the variogram model fit, which tracks the predictable change in shared community membership with distance. The vertical dashed line is the distance of spatial autocorrelation (range), which is the maximum distance, according to the model, at which similarity in community composition between samples is correlated (in this case, 240 m). The horizontal dashed line represents the 'nugget,' which is the proportion of the change in community composition not explained by the spatial model. The inset demonstrates that, past the autocorrelation distance, there is no predictable change in community composition with distance. Full size image Figure 2: Community-level spatial autocorrelation semivariogram. A semivariogram plot of the decay in community similarity (as measured by the UniFrac community dissimilarity metric on the y axis) with increasing distance between samples. A UniFrac value of 1 indicates no shared community members between two samples and a value of 0 indicates 100% shared community members. The solid line is the variogram model fit, which tracks the predictable change in shared community membership with distance. The vertical dashed line is the distance of spatial autocorrelation (range), which is the maximum distance, according to the model, at which similarity in community composition between samples is correlated (in this case, 240 m). The horizontal dashed line represents the 'nugget,' which is the proportion of the change in community composition not explained by the spatial model. The inset demonstrates that, past the autocorrelation distance, there is no predictable change in community composition with distance. Full size image To determine which, if any, subset of the bacterial community was changing across the landscape, we examined the spatial autocorrelation in genetic relatedness and relative abundance for major bacterial clades containing more than 100 sequences across all sampling sites (30 clades in all). Genetic relatedness and/or relative abundance of clades may account for community biogeographical patterns [5] ; however, across the high-alpine landscape, only the relative abundance of specific clades contributed to the community spatial pattern across the landscape (six clades, P ≤0.002, Moran's I for relative abundance, Supplementary Data ). These analyses show that high-alpine bacterial clades have distinct landscape-scale patterns in distribution, suggesting that bacterial clade relative abundance may be structured by patterns in biogeochemical parameters at the landscape scale. Habitat distribution modelling for bacterial clades Given the spatial patterning of microbial clades, we next determined which, if any, biogeochemical parameters underlie these patterns [4] . We used habitat distribution models [23] , [24] to analyse the habitat distributions of the 30 clades, in order to identify the major landscape-scale structuring factors. The models characterize the relationship between the relative abundance of bacterial clades and an extensive set of biogeochemical parameters across the landscape (21 different factors, including soil pH, plant cover, average annual snow depth, soil texture and extracellular enzyme activities, see Supplementary Data ). These independent analyses identified some of the same clades that spatial autocorrelation analyses did, including the Rhodospirillales, Rhizobiales, Acidobacteria G4 and Saprospirales, which were identified as having the highest levels of correlation with soil biogeochemical parameters ( Supplementary Data ). This approach yielded strong model fits with r 2 values between 0.53 and 0.62 ( Table 1 ), equivalent to the best r 2 values for models of plant and animal abundances at the landscape scale [23] , [24] . Table 1 Habitat-model spatial and biogeochemical components. Full size table To visualize how these clades are related to soil biogeochemical parameters, we mapped the habitat distributions for each of the three most abundant clades across the landscape ( Fig. 3 ); each mapped model describes the relative abundance of a clade on the basis of its response to the biogeochemical parameters at any one location in combination with a Kriged [25] spatial component that is a proxy for the influence of unmeasured biogeochemical parameters. In addition, out of the 21 biogeochemical parameters measured, we identified three parameters as the primary factors shaping microbial distribution in this environment ( Table 2 ). These parameters were soil pH, snow depth and forb abundance (forbs are broadleaved flowering plants, not grasses). Snow depth and plant abundance are known drivers of landscape structure in this extreme alpine environment [20] , [21] , [22] , and interact in that snow depth can control plant abundance in this system. In contrast, soil pH did not have a large interaction with other model variables, which suggests that pH measures a separate landscape process such as the composition of bedrock weathering products [26] . In addition, pH was the only model variable that showed a strong effect on the distribution of all four clades, which is in agreement with previous studies at continental scales [11] , [12] , [14] , and suggests that soil pH is an important driver of microbial community composition at both small and large scales. Although spatial studies have been conducted for microorganisms at many scales [6] , [7] , [8] , [9] , [10] , these models represent the first successful description of predictive habitat distributions for bacteria. 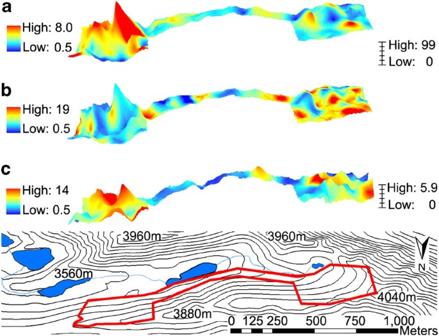Figure 3: Major clade habitat distribution maps. Maps of the sequence relative abundance as predicted by habitat distribution models for the three most abundant clades with a strong correlation with environmental variables. Each relative abundance map is depicted with four dimensions, the length and width representing geographical space, the vertical dimension representing forb abundance for the upper two maps and soil pH for the bottom map (hash mark scale on the right) and colour representing the relative abundance of each of the clades (scale on left, red=high; blue=low). The clades are (a) Rhizobiales, (b) Rhodospirillales and (c) Acidobacteria G4. The clade with the fourth highest relative abundance, the Saprospirales, had a distribution very similar to that of the Acidobacteria G4 and is not shown. The maps were created by cokriging25, an interpolation method that uses the 85 relative abundance measurements in combination with the environmental predictors from our model at all 160 sample locations to create a continuous map of relative abundance in the sampling area. The bottom topographic map shows the two-dimensional extent of the landscape. Figure 3: Major clade habitat distribution maps. Maps of the sequence relative abundance as predicted by habitat distribution models for the three most abundant clades with a strong correlation with environmental variables. Each relative abundance map is depicted with four dimensions, the length and width representing geographical space, the vertical dimension representing forb abundance for the upper two maps and soil pH for the bottom map (hash mark scale on the right) and colour representing the relative abundance of each of the clades (scale on left, red=high; blue=low). The clades are ( a ) Rhizobiales, ( b ) Rhodospirillales and ( c ) Acidobacteria G4. The clade with the fourth highest relative abundance, the Saprospirales, had a distribution very similar to that of the Acidobacteria G4 and is not shown. The maps were created by cokriging [25] , an interpolation method that uses the 85 relative abundance measurements in combination with the environmental predictors from our model at all 160 sample locations to create a continuous map of relative abundance in the sampling area. The bottom topographic map shows the two-dimensional extent of the landscape. Full size image Table 2 Landscape and global habitat distribution model coefficients. Full size table The predicted ecological niches based on our habitat distribution models confirm what is already known about some groups and suggest an unexpected dominance and new niche for another large group of bacteria. For example, the Rhizobiales are known plant root symbionts [27] ; hence it was not a surprise that their relative abundance was most highly correlated with plant abundance across the landscape. In contrast, our results pointed to the unexpected importance of the Rhodospirillales (our most abundant clade) across this alpine landscape. These organisms are mostly found in aquatic habitats where many of them fill a phototrophic niche, although they have extreme metabolic versatility encompassing photoheterotrophic, chemoorganotrophic and photoautotrophic lifestyles [28] . Although pH was the best predictor of the relative abundance of Rhodospirillales, the mechanism of this control for this group and for broader groups of microorganisms remains unknown [11] , [12] . However, although we do not yet know the Rhodospirillales' function in high-alpine soils, their negative correlation with plant abundance (the next strongest correlate) may indicate that they are outcompeted for light by plants in the alpine landscape and may be previously undocumented phototrophs in this environment. Rhodospirillales negatively correlated with soil nutrients and total microbial biomass as well ( Supplementary Data ), which, in combination with their metabolic versatility, suggests that these alpine microorganisms are well adapted to extremely oligotrophic areas. Regardless of their exact function, this is the first report of the widespread occurrence of Rhodospirillales in soil and we would not have predicted their importance across large expanses of the alpine landscape without detailed models of their habitat distribution. Global-scale predictive power of habitat distribution models To estimate global-scale applicability of bacterial habitat models to geographically separate high-elevation environments, we constructed Sanger clone libraries from six samples in each of four of the highest mountain ranges on Earth. These locations represent tests of our models against the extreme environmental limits of high-alpine systems (newly deglaciated soils near Mt Denali, late-melting snowbanks near the continental divide in the Colorado Rockies and alpine deserts in the high Andes and Himalayas; Supplementary Table S1 ). Taken together, the four clades identified in our pyrosequencing study made up a significant portion of the Sanger library microbial community in most of our sites, representing 26% of all bacteria in the Colorado Rockies, Himalayas and Alaskan range, but only 8% in the most extreme site, the high Andes. Our habitat distribution models correctly predicted the relative abundance of the four major clades from our pyrosequencing study across the entire global data set ( Fig. 4 ). The models in which the biogeochemical variables closely matched the Colorado Rockies environment had the highest predictive power; however, the models did not fit as well in areas with extreme differences in environment. In our most extreme global location, that is, the volcanic soils of the high Andes with almost no snowpack and no plant cover, the Rhodospirillales were, predictably, the group with the highest relative abundance, whereas the other three groups were absent or had very low relative abundances. This suggests that, although extreme habitats result in lower accuracy of habitat modelling for alpine bacteria, these same major clades are predictable in their importance globally. This conclusion is supported by our recent findings that fungal communities are very similar in plant-free soils of the Rocky Mountains, Himalayas and Antarctica [29] . Thus, high elevation and high latitude environments seem to harbour globally distributed microbial clades and are proving to be ideal environments to test hypotheses about the biogeography of soil microbial community diversity and function. 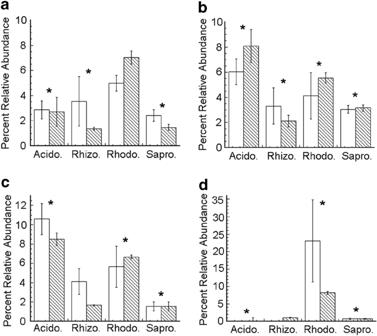Figure 4: Major clade global-scale abundances and model predictions. The relative abundance of Colorado's four major clades across high-alpine soils at a global scale (Acido, Acidobacteria G4; Rhizo, Rhizobiales; Rhodo, Rhodospirillales; and Sapro, Saprospirales; a, Rocky Mountains; b, Alaska Range; c, Himalayas; and d, Andes). Actual relative abundance: open bars; predictive habitat model relative abundances: shaded bars; error bars represent standard error; *indicates nonsignificant difference between actual and predicted (t-test,n= 6,P>0.05). Ordinary Least Squares (OLS) predictive habitat models using a restricted parameter set (see model parameters,Table 2). Acidobacteria G4 and Saprospirales had significant correlation between residuals (predicted relative abundance−actual relative abundance) and environmental variables, and are error corrected using OLS to predict residual error. Sanger relative abundances were rescaled because of the previously described biases in Sanger versus pyrosequencing14,41. Figure 4: Major clade global-scale abundances and model predictions. The relative abundance of Colorado's four major clades across high-alpine soils at a global scale (Acido, Acidobacteria G4; Rhizo, Rhizobiales; Rhodo, Rhodospirillales; and Sapro, Saprospirales; a, Rocky Mountains; b, Alaska Range; c, Himalayas; and d, Andes). Actual relative abundance: open bars; predictive habitat model relative abundances: shaded bars; error bars represent standard error; *indicates nonsignificant difference between actual and predicted ( t -test, n = 6, P >0.05). Ordinary Least Squares (OLS) predictive habitat models using a restricted parameter set (see model parameters, Table 2 ). Acidobacteria G4 and Saprospirales had significant correlation between residuals (predicted relative abundance−actual relative abundance) and environmental variables, and are error corrected using OLS to predict residual error. Sanger relative abundances were rescaled because of the previously described biases in Sanger versus pyrosequencing [14] , [41] . Full size image Although other studies have shown that (1) spatial patterns exist in soil microorganisms [6] , [7] and (2) steep gradients in soil chemistry are correlated with phylum-level changes in microbial community composition [20] , [21] , our study is the first to successfully link spatial autocorrelation in microbial communities to the distribution of individual clades and to demonstrate that these distributions can be modelled with strong predictive power across the landscape and the globe. We did this by examining the relationship between narrowly defined bacterial clades and soil environmental and biogeochemical patterns, which affords greater power to identify ecological patterns than do previous operational taxonomic unit diversity [6] , [7] or phylum level [11] , [12] studies. By examining narrowly defined clades, we were able to provide the first environmental-sequencing-based description of ecological niches for bacteria and identify unexpectedly important bacterial clades such as the Rhodospirillales. In addition, the groups that showed the highest level of spatial structuring across the landscape have predictable distributions in high-elevation soils across the globe, suggesting that these groups are easily dispersed and are of significant importance to alpine biogeochemistry and bacterial community dynamics. These findings are evidence that soil microorganisms are not homogeneously distributed across landscapes but rather occur in patches the composition of which is related to the landscape distribution of biogeochemical properties. This approach is uniquely ecosystem focused and greatly expands our ability to link changes in community diversity with the relative abundance of individual bacterial clades and understand the ecology of soil organisms across the landscape and the Earth. Sampling scheme A total of 160 soil samples were collected from a continuous landscape on the south side of the Green Lakes Valley Watershed (GLV), CO, USA. We sampled a distinct and well-defined landscape unit within the GLV that is bound on the east by the tundra, on the south by alpine lakes, glaciers and meadows, on the west by the continental divide and on the north by steep cliffs. There is a large cliff face in the centre of our landscape, along the base of which exists a narrow 75 m wide corridor that connects the upper and lower parts of the landscape ( Fig. 1 ). The sampled landscape is composed of a matrix of block slope, late-melting snow banks overlaying unvegetated gravel soils, fellfields and small patches of vegetation [20] , [22] , [30] . However, even in the most developed soils, the soil texture is high in sand content and the total soil depth is minimal. The valley receives the majority of its precipitation during winter months [14] and many snow banks do not completely melt until late July/early August. Our sampling was conducted from 4–8 September 2007 in order to minimize the effects of localized variation in soil water because of snowmelt subsidies. The main goal of our sampling effort was to construct spatially explicit landscape models. Such models require a subset of samples to be collected at a small enough scale in order to establish a baseline for the spatial autocorrelation [31] . A preliminary study of GLV Watershed soils [22] spanning sampling distances from 10 cm to 1 km was used to determine an optimum sampling interval of 50 m. However, to generate accurate spatial models, we selected three locations for smaller spaced sampling, which was performed in a 5 m grid over 30 m×30 m plots. At each sampling location, a 10 cm diameter section of soil to 4 cm depth in the approximate centre of the soil patch closest to the predetermined grid point was mixed and ∼ 75 g placed in a sterile conical tube. The location of each sampling point was recorded with a Garmine eTrex Vista gps unit (Garmin International). Soil samples were stored at 4 °C for a maximum of 1 week while soil-dissolved organic carbon and total dissolved nitrogen measurements were taken. Afterwards, soils were stored at −20 °C until processing. Soils for soil texture analysis were collected from each location in September 2008. Sequencing and biogeochemical measurements Microbial diversity data for the GLV samples were obtained by pyrosequencing 85 randomly selected samples (out of 160 total) ( Fig. 1 ) for the 16S gene using the method of Fierer et al . [32] and resulting in 16,894 sequences with an average length of 230 nucleotides. Dissolved organic C/N and microbial biomass C/N were determined, and analysis of extracellular enzymes N -aceytalglucosaminase, β-glucosidase, α-glucosidase, β-xylase, cellobiosidase, leucine amino-peptidase, organic phosphatase and lignin oxidase/peroxidase was performed using the methods of Weintraub et al . [33] Soil pH was measured after the addition of 2 ml water to 2 g soil and shaking for 1 h. Soil water content and soil water holding capacity were measured gravimetrically. Soil texture (clay/sand/silt) was measured by South Dakota Soil Laboratory (South Dakota State University, Brookings, SD, USA). Plant diversity and abundance were measured by identifying and recording all vascular plants within a 1 m radius of a sampling location. Snow depth values at each point were obtained by averaging the snowpack depth from the kriging interpolations of snow surveys in the GLV from 1997 to 2003 (Niwot LTER database, http://culter.colorado.edu/exec/Database/gis_layer_query.cgi ). Degree of slope was calculated on the basis of a 10 m digital elevation model also available from the Niwot LTER website. Phylogenetics and habitat modelling Clades were defined by selecting all nodes on the full community tree that aggregated at least 100 sequences (12,303 sequences were obtained, an average of 145 sequences per sample). Semivariograms, correlation matrices and correlation significance tests were performed in R [34] (version 2.8.1, 22 December 2008, The R Foundation for Statistical Computing http://www.r-project.org/index.html ) with the aid of the spatial statistics add-on package geoR. Semivarogram models were fit in R for a spherical model [25] using a Nelder–Mead nonlinear algorithm [35] . Mantel tests for spatial autocorrelation models [36] were evaluated from 0 m to the modelled distance of autocorrelation for each semivariogram in R using the statistics add-on package ade4 using 1,000 iterations. Moran's I -tests for spatial autocorrelation [37] in clade relative abundance were conducted in R using in spatial statistics add-on package ape. Clade habitat distribution models were constructed in the Spatial Analyses in Macroecology (SAM [38] ) programme using the Akaike information criterion [39] to select environmental variables and a generalized least squares spatial partial regression to add the spatial component. Maps were generated in ArcGIS 9.3 (ESRI) using cokriging of the relative abundance for each clade on 85 sequenced samples, in combination with the three most significant environmental variables in each habitat distribution model for all 160 samples [25] . Cokriging was chosen to generate the maps of the distribution of the clades because it creates a continuous map surface using a linear least squares model similar to our SAM models and has an estimation error that is dependent on the spatial autocorrelation distance for the variable of interest (relative abundance). Thus, the error is relatively low for estimations at distances less that the clade's autocorrelation distance from sample locations [25] . Global-scale sampling and analysis For the global biogeographical analysis, we collected six samples from each of four sites during the regional dry season using the same methods as for the main Colorado Rocky Mountains data set ( Table 2 ). The sites were GLV, Denali National Park & Preserve, AK, USA (DNP&P); Annapurna Conservation Area, Nepal; and Llullaillaco Volcano, Argentina. Samples from outside the United States were frozen in the field, kept frozen during transportation from the field, shipped frozen through express airmail and stored at −20 °C until processed. For each sample, DNA was extracted and Sanger clone libraries for the 16S gene were constructed according to the methods of Freeman et al . [29] , resulting in 3,429 sequences. A restricted set of biogeochemical properties was measured for each site using the same methods as for the primary Colorado data set (soil water content, soil water holding capacity, all eight extracellular enzymes, forb abundance, soil pH, microbial biomass C&N, total dissolved nitrogen and dissolved organic carbon). After the initial (Niwot) models were used to predict the relative abundance, we looked for additional predictor variables that showed a broader range of variation and had significant correlation with the residuals (predicted relative abundance—actual relative abundance) on the global scale. Clades with significant correlation between residuals and environmental variables (Acidobacteria G4 and Saprospirales) were error corrected using ordinary least squares regression to predict residual error. The reason that these variables were not adequately weighted in the original model is because the DNP&P and Annapurna soils are formed from calcareous shale bedrock, whereas the GLV (and Llullaillaco) site is formed from igneous bedrock. The shales of the DNP&P and Annapurna sites create soils with a significantly more basic pH (7.5 versus 4.5, t -test, P <0.001). This difference in soil pH is known to have a significant effect on extracellular enzyme activity, particularly for leucine peptidase, which, similar to most peptidases, has its activity optimum in basic pH solutions [40] (11 versus 0.01, t -test, P <0.001). In addition, DNP&P and Annapurna soils had lower water holding capacities than found in the main GLV data set (0.27 versus 0.46, t -test, P =0.016). As a result, the habitat models for Acidobacteria G4 and Saprospirales are error corrected by adding leucine amino-peptidase activity, which was only appreciably active at pH>7, as a model parameter, and reweighting the contribution of water holding capacity and soil pH. In essence, we had to broaden the range of predictability of the models once we had data across a wider range of pH values. Relative abundances were rescaled for Figure 4 because of a bias in Sanger versus pyrosequencing that we observed in the six samples from Colorado that were analysed using both sequencing approaches (Sanger relative abundance * factor: Acidobacteria G4, *0.667; Rhizobilaes, *2.85; Rhodospirillales, *6.54; Saprospirales, *0.204; raw relative abundances are given in Supplementary Table S2 ). Similar effects have been observed in previous comparisons of Sanger versus pryosequencing, although the cause of this bias is still the subject of debate [14] , [41] . However, the fact that these rough rescalings enabled the accurate prediction of Sanger relative abundances based on models of pryosquencing data suggests that these biases are consistent across samples and, given absolute abundance estimates derived from a method such as fluorescence in situ hybridization, similar types of correction factors could be used in future to estimate actual abundances of microbial clades in soil samples. For additional details on DNA extraction, sequence processing and phylogenetic determination, see Supplementary Methods . Sequences are available at the Alpine Microbial Observatory Website: http://amo.colorado.edu/database.html Sequences have been deposited in NCBI's Genbank database under accession numbers HM780503 - HM797396 . How to cite this article: King, A. J. et al . Biogeography and habitat modelling of high-alpine bacteria. Nat. Commun. 1:53 doi: 10.1038/ncomms1055 (2010).